Remnants of an ancient forest provide ecological context for Early Miocene fossil apes The lineage of apes and humans (Hominoidea) evolved and radiated across Afro-Arabia in the early Neogene during a time of global climatic changes and ongoing tectonic processes that formed the East African Rift. These changes probably created highly variable environments and introduced selective pressures influencing the diversification of early apes. However, interpreting the connection between environmental dynamics and adaptive evolution is hampered by difficulties in locating taxa within specific ecological contexts: time-averaged or reworked deposits may not faithfully represent individual palaeohabitats. Here we present multiproxy evidence from Early Miocene deposits on Rusinga Island, Kenya, which directly ties the early ape Proconsul to a widespread, dense, multistoried, closed-canopy tropical seasonal forest set in a warm and relatively wet, local climate. These results underscore the importance of forested environments in the evolution of early apes. The origin and early diversification of crown catarrhines (cercopithecoids and hominoids) took place in Afro-Arabia from 28 to 18 million years ago [1] and is well documented in Early Miocene deposits of East Africa by a diversity of stem catarrhines, rare fossil monkeys and the appearance of the first fossil apes [2] . Rusinga Island, Kenya, is a key source of palaeobiological information from the end of this period, preserving at least two fossil ape genera and two stem catarrhines among more than 100 vertebrate species and diverse invertebrate and plant fossils. The majority of these fossils are from the Hiwegi Formation, although specimens can be found throughout most of the ~300-m thick Rusinga Group strata ( Fig. 1 ). 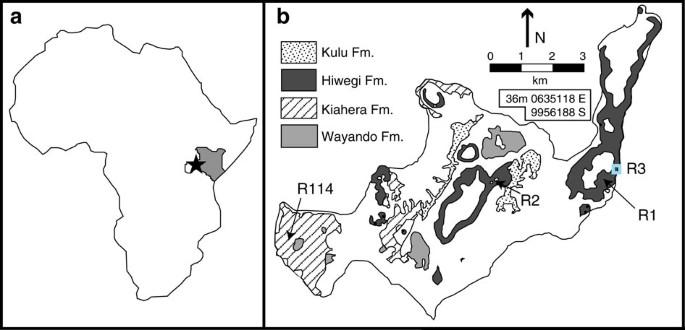Figure 1: Location and geological map of Rusinga Island. (a) Map of Africa with the location of Rusinga Island indicated by the black star. (b) Geological map of Rusinga Island on eastern edge of Lake Victoria showing important localities and Miocene stratigraphy. Blue box denotes the location of the R3 locality. Figure 1: Location and geological map of Rusinga Island. ( a ) Map of Africa with the location of Rusinga Island indicated by the black star. ( b ) Geological map of Rusinga Island on eastern edge of Lake Victoria showing important localities and Miocene stratigraphy. Blue box denotes the location of the R3 locality. Full size image Similar to most East African fossil assemblages, historical collections from Rusinga primarily represent time-averaged and reworked accumulations derived from multiple fossiliferous strata. Although these time-averaged interpretations are important for assessing large-scale palaeobiological trends, such as the presence of specific mammalian taxa, the temporal and spatial conflation of fossil assemblages presents significant challenges for reconstructing individual habitats and for determining habitat preferences of individual species and species assemblages. Furthermore, most palaeoenvironmental interpretations for Rusinga, which are based on these time-averaged and reworked assemblages, probably sample multiple palaeoenvironments. This may explain, in part, contradictory interpretations for Rusinga’s palaeohabitats, ranging from closed forested systems to mixed habitats of open and closed environments to open woodland or grassland environments [3] , [4] , [5] , [6] , [7] , [8] , [9] , [10] , as well as explain a bias towards findings of ‘mixed habitats’. A few studies on Rusinga have assessed the palaeoenvironment using restricted stratigraphic intervals [4] , [8] , [9] , [11] , but in most cases these strata are not directly associated with fossil mammals [4] , [8] , [11] . One exception is the study of ‘Whitworth’s Pothole’ at the R114 locality in the Kiahera Formation ( Fig. 1 ), which assessed fossils that probably accumulated by a carnivorous mammal within an infilled tree trunk [9] . The presence of the fossil-bearing infilled tree trunk, plus other circular deposits in this same area that were also interpreted to represent infilled tree trunks, were used to infer that R114 sampled a forested environment [9] . However, this supposition could not be properly tested. Approximately 4 m of volcanic ash buried the infilled tree trunks preventing an assessment of the palaeosol within which the trees grew and of the stratigraphic correlation of the tree trunks across the paleolandscape. Likewise, no analyses of the tree trunk distribution or density were performed. Thus, it is not possible to determine whether the R114 site represented a forested environment or a stand of trees within a more open woodland or grassland environment, or even a time-equivalent assemblage. Our recent discovery on Rusinga of an expansive fossil forest system, preserved within a single palaeosol and associated with vertebrate, invertebrate and fossil leaf specimens, enables us for the first time to develop a high-resolution, multi-proxy reconstruction of a complete, individual fossil ape habitat dating to ~18 million years ago [12] , [13] . Palaeopedology Within the Kibanga Member of the Hiwegi Formation ( Fig. 2 ), 29 tree stump casts, composed of red coarse sand to granule-size tephra and ash, were discovered at Rusinga’s R3 locality and mapped across the landscape using a differential global positioning system and total station ( Fig. 3a ). Twenty-seven of these were measurable and exhibited diameters ranging from 18 to 160 cm ( Supplementary Table 1 ). In the same horizon, distinct, calcified root casts ranging from 1.0 to 49.5 cm in diameter were preserved for up to 5 m away from their respective stumps. The root casts show branching patterns, have traceable attachments to the stump casts and occur at many different depths through the palaeosol ( Fig. 3 ). In some cases, multiple root casts branch away from areas without exposed stumps or extend into areas where the palaeosol horizon is eroded away, suggesting the former presence of additional stump casts across the landscape. When thin-sectioned, primary structures including relict xylem and phloem were observed ( Fig. 3e ). The horizontal nature of the roots, combined with the low-Mg calcite cementation of final pore space in the palaeosol, suggests a shallow water table, explaining the co-occurrence of stumps and roots in the same horizon. 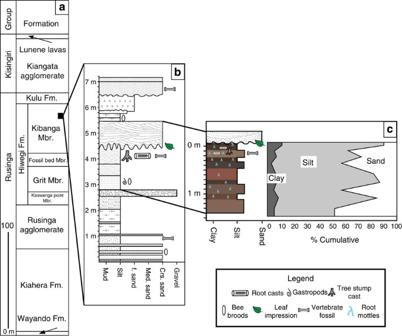Figure 2: Stratigraphy of Miocene deposits on Rusinga Island and at the R3 fossil locality. (a) Generalized stratigraphy of Miocene deposits on Rusinga Island68. (b) Stratigraphy of the R3 locality. (c) R3 type paleosol (Table 2) field description and grain size generated from a mastersizer grain size analyzer. Figure 2: Stratigraphy of Miocene deposits on Rusinga Island and at the R3 fossil locality. ( a ) Generalized stratigraphy of Miocene deposits on Rusinga Island [68] . ( b ) Stratigraphy of the R3 locality. ( c ) R3 type paleosol ( Table 2 ) field description and grain size generated from a mastersizer grain size analyzer. 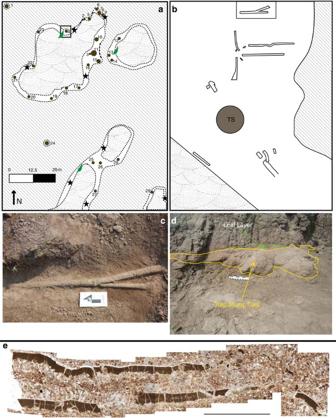Figure 3: Distribution and images of tree stump and root casts across the forest paleosol horizon at R3. (a) Detailed map showing distribution of tree stump casts (circles) at R3 site. Diameter of circles is directly proportional to the diameter of the tree stump casts. Stars indicate measured paleosol profiles. Leaf symbols represent quarries where fossil leaves were excavated from superjacent sandstone horizon. Box indicates the location of the calcite-cemented root casts, tree stump casts and palaeosol excavated and illustrated inb. (b) Drawing depicting spatial relationship of one tree stump cast (TS) and root complex. (c) Close-up photograph of an excavated root showing branching behavior (15 cm scale). (d) Photograph of excavated tree stump cast (yellow) directly overlain by fossil leaf layer (green) (15 cm scale). (e) Thin-section photomicrographs of one small root cast (plane-polarized light). Initial root morphology affected preservation, manifested by dark band (xylem) and relict interior cell (phloem) structure (scale bar: 1 cm). Full size image Figure 3: Distribution and images of tree stump and root casts across the forest paleosol horizon at R3. ( a ) Detailed map showing distribution of tree stump casts (circles) at R3 site. Diameter of circles is directly proportional to the diameter of the tree stump casts. Stars indicate measured paleosol profiles. Leaf symbols represent quarries where fossil leaves were excavated from superjacent sandstone horizon. Box indicates the location of the calcite-cemented root casts, tree stump casts and palaeosol excavated and illustrated in b . ( b ) Drawing depicting spatial relationship of one tree stump cast (TS) and root complex. ( c ) Close-up photograph of an excavated root showing branching behavior (15 cm scale). ( d ) Photograph of excavated tree stump cast (yellow) directly overlain by fossil leaf layer (green) (15 cm scale). ( e ) Thin-section photomicrographs of one small root cast (plane-polarized light). Initial root morphology affected preservation, manifested by dark band (xylem) and relict interior cell (phloem) structure (scale bar: 1 cm). Full size image Trees were preserved in a brown, friable palaeosol composed mostly of sand-sized grains, with soil peds ranging from massive to weak angular blocky. The palaeosol shows weak paedogenic development (Inceptisols [14] or Protosols [15] ) and includes pressure faces, and evidence of aggradation of at least four fining-upwards successions ( Fig. 2c ). On the basis of micromorphologic evidence of illuviated clay and moderately weathered pyroxene, amphibole, feldspar and fragments of volcanic rock, the landscape is interpreted to have been stable for tens to a few hundred years, consistent with weak geochemical differentiation [16] . Clay mineralogy is dominantly composed of illite and smectite with minor quartz and calcite, which results from incomplete weathering of volcanic detritus [16] . Macromorphological features, including incipient pressure faces in the soil, suggest that precipitation was likely to be seasonal, with a distinct wet and dry period. Using time-correlative strata, we were able to identify and map the same palaeosol and additional stump casts and root systems above fossil locality R1 and at locality R2, the latter of which is ~4.3 km away ( Fig. 1 ). Correlation of the palaeosol among these localities indicates that the forest was widespread and possibly continuous across the area. There is no evidence within the palaeosol for fluvial processes, suggesting that the vertebrate assemblage located within does not represent a riverine deposit. Furthermore, the palaeosol is truncated by a coarse-grained sandstone lacking vertebrate remains, which indicates rapid burial of the fossil-bearing horizon ( Fig. 2 ). Forestry Reconstructing the forest structure using the basal area and density of stump casts places the R3 forest among the densest closed-canopy forests worldwide, irrespective of geography, climate, dominant tree family or canopy architecture ( Table 1 ). Although forests have considerable structural heterogeneity at grain sizes of 20–50 m, comparable to the sampled area at Rusinga [17] , the 95th percentile densities and basal areas in modern heterogeneous forests are twice the mean values (maxima are typically three times mean values [18] ). Therefore, even if the sampled area on Rusinga had been at the 95th percentile of tree density and basal area for the fossil forest, overall tree densities and basal areas would have been no lower than half the calculated values ( Table 1 , ‘Rusinga lower bound’). This abundance and proximity of tree stump casts of varying diameters at R3 implies that the forest would have comprised trees with interlocking or overlapping crowns. Table 1 Comparison of Rusinga Island forest reconstruction to modern forests. Full size table Palaeobotany In addition to tree and root casts, abundant well-preserved leaf fossils were found within a thin mudstone lens at the base of a coarse-grained sandstone layer overlying the palaeosol ( Figs 2 , 3 , 4 , 5 ). Leaves were found in the same stratigraphic position across R3, suggesting that they represent minimally transported forest floor leaf litter. Although the preserved leaves cannot be directly related to the underlying palaeoforest layer, their superjacent stratigraphic position suggests that they represent a similar, if not identical, environment. The flora, comprising 29 morphotypes representing 27 dicotyledonous (dicot) angiosperms and 2 monocotyledonous angiosperms, was dominated by species with long-lived leaves ( Figs 4 , 5 and Supplementary Table 2 ). Eighty-nine percent of the dicot morphotypes are entire margined. Our preliminary morphotyping and field assessment indicates that there were differences in morphotype occurrences and abundance across the R3 locality. Leaf litter reliably preserves the spatial distribution and heterogeneity of the plants within modern forests [19] ; thus, the differences between quarries may reflect variability in spatial distribution of tree species across the landscape. 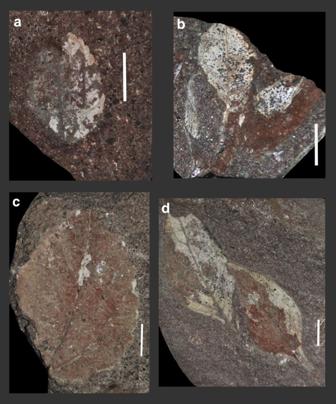Figure 4: Common dicotyledonous morphotypes from R3 fossil leaf layer. (a) Morphotype 15 showing ovate shape, three basal veins, prominent basal agrophics and teeth; (b) morphotype 20 showing three palmate lobes, actinodromous primary venation and highly ascending, eucamptodromous venation; (c) morphotype 4 showing ovate shape, pinnate primary venation with basal agrophic, brochidodromous secondary venation and opposite percurrent tertiary venation; (d) morphotype 1 showing a compound leaf with pinnate primary venation, eucamptodromous secondaries, a stout petiole and a prominently acute base. Scale bar in all photographs is 1 cm. Figure 4: Common dicotyledonous morphotypes from R3 fossil leaf layer. ( a ) Morphotype 15 showing ovate shape, three basal veins, prominent basal agrophics and teeth; ( b ) morphotype 20 showing three palmate lobes, actinodromous primary venation and highly ascending, eucamptodromous venation; ( c ) morphotype 4 showing ovate shape, pinnate primary venation with basal agrophic, brochidodromous secondary venation and opposite percurrent tertiary venation; ( d ) morphotype 1 showing a compound leaf with pinnate primary venation, eucamptodromous secondaries, a stout petiole and a prominently acute base. Scale bar in all photographs is 1 cm. 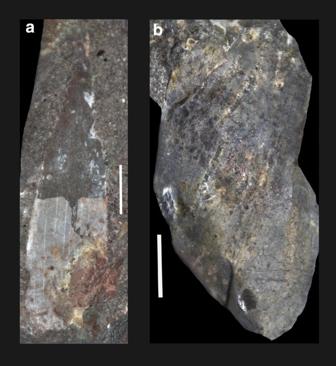Figure 5: Monocotyledonous morphotypes from R3 fossil leaf layer. (a) Morphotype 2 showing two orders of parallel veins, primary veins very prominent, seven secondary veins between primary veins, an acute apex and an elliptic shape; (b) morphotype 30 showing two orders of parallel veins and five secondary veins between primary veins. Both scale bars are 1 cm. Full size image Figure 5: Monocotyledonous morphotypes from R3 fossil leaf layer. ( a ) Morphotype 2 showing two orders of parallel veins, primary veins very prominent, seven secondary veins between primary veins, an acute apex and an elliptic shape; ( b ) morphotype 30 showing two orders of parallel veins and five secondary veins between primary veins. Both scale bars are 1 cm. Full size image Leaf mass per area ( M A ) of the flora suggests the forest comprises predominantly evergreen taxa, but deciduous taxa with short-lived leaves would have also been an important component (site mean M A =125.0, +114.0, −57.9 gm −2 , errors represent 95% prediction interval, range=70–196 gm −2 , n =16; Supplementary Table 2 ). The average leaf area (site mean=7.83 log e mm 2 , range=6.0–9.1 log e mm 2 , n =24; Supplementary Table 2 ) and the proportional abundance of large leaves (100% ≥ microphyll sized; Supplementary Table 2 ) is characteristic of closed forested environments [20] . Palaeoclimate estimates from the flora suggest mean annual temperature and mean annual precipitation ranging between 22.6 °C and 34.5 °C, and 1,394 mm and 2,618 mm, respectively. Wet-month precipitation estimates suggest that relatively little precipitation would have fallen during the dry season ( Supplementary Table 3 ). Considering both leaf physiognomy and palaeoclimate estimates, the R3 flora compares most favourably with modern tropical seasonal forests, such as those that support communities of medium- to large-bodied primates (for example, Barro Colorado Island, Panama and Pasoh Forest Reserve, Malaysia) [21] , [22] ( Table 1 ). Vertebrate palaeontology There are at least three distinct terrestrial vertebrate horizons at R3 ( Fig. 2b ). The most fossiliferous of these is within the palaeosol interval. Surface collections and excavations conducted between 2011 and 2013 recovered ~400 fossils from the palaeosol layer ( Supplementary Table 4 ), including associated dental specimens of the early ape Proconsul ( Fig. 6 ). Four teeth (dI 1 , dC 1 , dP 4 and M 1 (unerupted)) attributed to a single individual of Proconsul heseloni ( Fig. 6 ) were discovered within the palaeosol interval next to one of the large stump casts. In addition, four partial skeletons of the catarrhine primate Dendropithecus macinnesi , found in 1950 at sublocality R3a [23] , can be directly tied to this forest habitat by lithostratigraphic correlation. Other primate taxa, including Limnopithecus and Nyanzapithecus , and the strepsirhine primates Komba and Progalago , have historically been surface collected at R3 (ref. 24 ; Supplementary Table 4 ), and many of these are likely to be derived from this forest interval, but a lack of detailed provenience information for these specimens prevents us from directly locating them within the palaeosol. 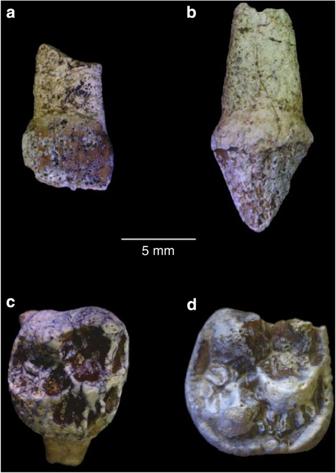Figure 6: Associated teeth from a specimen ofP. heselonifound in the forest palaeosol horizon. (a) Deciduous left I1(labial view); (b) deciduous left upper canine (lingual view); (c) deciduous left P4(occlusal view); and (d) left M1(occlusal view). Figure 6: Associated teeth from a specimen of P. heseloni found in the forest palaeosol horizon. ( a ) Deciduous left I 1 (labial view); ( b ) deciduous left upper canine (lingual view); ( c ) deciduous left P 4 (occlusal view); and ( d ) left M 1 (occlusal view). Full size image The non-primate fauna from R3 is also consistent with, although not diagnostic of, the presence of a closed-forest environment ( Supplementary Table 4 ). Viewed as a whole, the mixed historical collections from R3 include taxa representing both open and closed environments. However, the discovery by our team of an in situ gomphothere specimen ( cf. Archaeobelodon sp.) in a lower fossil horizon at R3 suggests that this older stratum might represent a more open interval [25] . Considering only specimens of known association with the forest palaeosol, we find no definitively open-adapted species ( Supplementary Table 4 ). Small ruminants (in particular Dorcatherium pigotti ), squirrels ( Vulcanisciurus ), anomalurid rodents, chalicotheres ( Butleria ) and snakes, all indicate a closed ecosystem. Other taxa (several rodent groups, macroscelids, tubulidentates, erinaceids, middle- to large-sized carnivores and non-specialized suids) are thought to have inhabited a variety of habitat types, including forests. The environmental preferences of springhare ( Megapedetes ) and cursorial large hyraxes ( Afrohyrax ) are currently unknown, and our discovery of these within this palaeosol indicates at least a capacity, if not necessarily a preference, for living in a closed ecosystem. The multiple lines of evidence presented herein provide direct evidence for the existence of widespread, closed forested environments in the Early Miocene on Rusinga Island. Our work, combined with previous environmental interpretations of more open environments [4] , [6] , indicates that Early Miocene palaeoenvironments on Rusinga were dynamic and varied through time. This in turn suggests that early apes lived in and had adaptations that allowed them to exploit both open and closed environments. Although Proconsul probably had a positional repertoire more similar to modern monkeys than apes, several of its features suggest more ape-like climbing and clambering behaviours, which is consistent with a phylogenetic position within the Hominoidea ( Fig. 7 ). A relatively long, strong hallux with a well-developed flexor hallucis longus muscle indicates powerful grasping capabilities that would have facilitated arboreal locomotion [26] , [27] . Likewise, a rounded humeral head and lateral trochlear ridge on the distal humerus suggest mobility at the shoulder and elbow, and joint stability across the range of pronation and supination [27] , [28] , [29] . Without the aid of a tail for balance [30] , this combination of forelimb anatomy and powerful grasping would have accommodated Proconsul ’s habitual use of arboreal supports within a closed forest [31] . Dendropithecus , although not as well-represented skeletally, also displays features indicative of climbing and even suspensory behaviours that are more easily interpreted in the context of a multistoried forest [2] . This generalized arboreal repertoire, widespread among Early and early Middle Miocene catarrhines, may have been important in much younger hominoid taxa, and has even been implicated in interpretations of the behaviour and locomotion of the basal hominin Ardipithecus ramidus [32] . 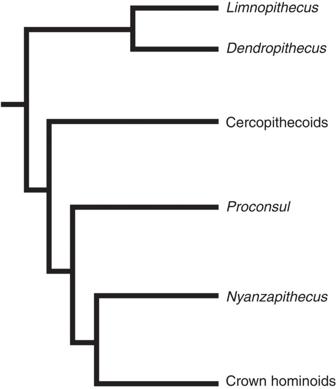Figure 7: Dendrogram, simplified from the cladistic analysis presented by Stevenset al.1, depicting the relationships of Rusinga’s catarrhine primates to crown catarrhine superfamilies. On the basis of that analysis, bothProconsulandNyanzapithecusgroup with the Hominoidea, whereasDendropithecusandLimnopithecusare stem catarrhines. Figure 7: Dendrogram, simplified from the cladistic analysis presented by Stevens et al. [1] , depicting the relationships of Rusinga’s catarrhine primates to crown catarrhine superfamilies. On the basis of that analysis, both Proconsul and Nyanzapithecus group with the Hominoidea, whereas Dendropithecus and Limnopithecus are stem catarrhines. Full size image Our results document the occurrence of primitive apes and many other fossil vertebrates within a widespread, dense, multistoried, closed-canopy forest; however, we note that the forest represents a restricted temporal interval within a much longer palaeoenvironmental history during the Early Miocene. Although associating this fossil assemblage within a well-characterized habitat is important for interpreting the evolutionary dynamics between mammal communities and their environments, fully resolving the adaptive significance of these animals will require similar associations across their temporal and geographic ranges. These taxa are known from several East African early Miocene sites [24] , suggesting that it is possible to directly assess temporal and spatial patterns of early primate evolution. Future research should emphasize multiproxy palaeoenvironmental reconstructions, particularly sampling other East African fossil localities, to document the impact of Early Miocene tectonic and climatic shifts on local ecosystems and their mammalian communities. Palaeopaedology Fieldwork at R3 was conducted in June and July of 2011. Palaeosols were trenched back 15–30 cm to remove surficial weathering before they were described using methods outlined for modern soils [33] and advised for palaeosols [34] , including description of ped shape, size, colour and texture of the palaeosol layers, and boundary conditions ( Table 2 ). Once described, each horizon was sampled for bulk geochemistry and clay mineralogy before being coated with polyester resin to stabilize the rock for thin-section analysis. Twenty-three samples were sent to Spectrum Petrographics, Inc. for thin-section preparation. Thin sections prepared from the palaeosol at R3 were examined using an Olympus BX51 research microscope equipped with a 12.5 Mpx digital camera. Thin sections were described using standard soil micromorphological terminology [35] , [36] , [37] , [38] . Table 2 Measured section description for type paleosol from the R3 fossil locality. Full size table Forestry On the basis of the distribution and spatial relationships of stump casts across the landscape, we were able to reconstruct forest structure and density. We inferred forest structure by comparing the landscape density and basal area of the stumps with data from that of modern forests. In our analyses, we took into account differences between stump diameter and traditional metrics for tree size and the potential for sampling effects, the loss of smaller trees during ash fall and fossilization, and the likelihood that preserved stumps represent living trees, snags and/or stumps in the pre-eruption forest. To establish equivalency in density and basal area with contemporaneous forests, we first used existing allometric relations to convert between stump diameter and diameter at breast height (DBH; 1.3 m above the ground), assuming that the preserved tree bases represented stumps 5 cm high. Allometric relationships between stump heights and DBH do not exist for African tree species in the same diameter range as the Rusinga Island data. Therefore, we selected allometric equations derived from contemporaneous data for representatives of three plant families with appropriate diameter ranges: Pinaceae, Cupressaceae and Salicaceae [39] . The allometric equations represent a range of tree tapers, with the equation for Thuja plicata (Cupressaceae) yielding the most conservative (smallest) value of DBH. The 27 stumps had diameters ranging from 18 to 160 cm, yielding DBH values from 11 to 96 cm ( Table 1 ). However, owing to the difficulty in judging uniform preservation of smaller trees following volcanic eruptions [40] , and also to concentrate on those trees providing sufficient vertical structure for vertebrate habitat, we limited our analysis to trees ≥30 cm DBH (21 trees). We reduced the estimates of tree density and basal area of the R3 stumps by an approximation for the ratio of live trees (or basal area) to the sum of live trees, snags and stumps from a forest with long residence time for dead trees because the fossilized stump casts could represent living trees, snags or stumps, and we assumed that dead trees played a limited role in usable forest structure [18] . The total area used as a basis of developing forest estimates was 930.11 m 2 , comparable to other palaeoreconstructions [41] . We compared the calculated values of density and basal area for trees ≥30 cm DBH and for trees ≥60 cm DBH with those of contemporary forests taken from the Smithsonian Center for Tropical Forest Science plot network [18] , [21] , [42] . Palaeobotany Fossil leaves were collected from a series of thin mudstone lenses at the base of the coarse-grained sandstone layer overlying the forested palaeosol horizon. Fossil leaves were stratigraphically correlated across the R3 locality. Fossils were collected from three quarries at R3 ( Fig. 3a ). Collection occurred by removing large blocks of matrix split along bedding planes to expose the leaves using chisels and rock hammers. Each fossil leaf quarry covered a few square metres because the fossiliferous layers were relatively thin (~5–20 cm thick). Fossil leaves were collected selectively from each quarry. In the field, specimens were lumped together into preliminary morphotype categories based on their morphological characteristics. More than 350 specimens were examined during quarrying. After examination in the field, 160 voucher specimens that were >25% complete or that had unique morphological characteristics, such as teeth or well-preserved higher-order venation, were collected. At the National Museums of Kenya, Nairobi, our field identifications were assessed and all identifiable voucher specimens were assigned to a morphotype ( Supplementary Table 2 ). Morphotypes are morphologically distinct groups of specimens that have no taxonomic status, but often reflect biological species [43] , [44] . All voucher specimens were photographed and used in our palaeoclimate analyses. The fossils are currently housed at the National Museums of Kenya. Mean annual temperature was estimated using leaf margin analysis models [22] , [45] , [46] , [47] , and mean annual precipitation was estimated using leaf area analysis equations [22] , [48] , [49] , [50] . Wet-month precipitation, which is the total precipitation for all months exceeding 50 mm of rainfall, was estimated using the leaf area analysis regression of Jacobs and Herendeen [50] ( Supplementary Table 3 ). Leaf mass per area ( M A ) and leaf life span was estimated using the methods of Royer et al. [51] (model E: log[M A ]=3.070+0.382[log[petiole width 2 /leaf area]]; Supplementary Table 3 ). Vertebrate palaeontology Specimens used in this study were primarily surface collected with some limited to excavation from 2008 to 2013 ( Supplementary Table 4 ). Fossils collected from 2011 to 2013 were mapped using a differential global positioning system and total station to determine their precise location. All fossils were directly related to the R3 stratigraphy to determine their stratigraphic position ( Fig. 3b ). Catarrhine phylogeny Figure 7 introduces a working hypothesis for the relationships of Rusinga’s catarrhine primates to the crown catarrhine clades of cercopithecoids (Old World monkeys) and hominoids (apes and humans). This simplified dendrogram is based on the most recent cladistic analysis of these and other related taxa [1] . Although this topology is probably not stable— Nyanzapithecus vancouveringorum and Limnopithecus legetet in particular are not well known from skeletal elements beyond the dentition—the tree provides an evolutionary context for interpreting the discovery of two of these taxa, Proconsul and Dendropithecus , within the forest at Rusinga site R3. Here we follow the majority of researchers who place Proconsul within the Hominoidea, typically as a stem ape [1] , [2] , [26] , [27] , [29] , [31] . This genus has long provided the basic model for the anatomy of the earliest apes. However, a small number of workers—led by Harrison [2] , [52] —maintain that Proconsul originated before the differentiation of crown catarrhines and support this claim with several morphological characteristics. The discovery in Morotopithecus of features suggestive of vertical positional behaviours also provides an alternate model of what early apes might have looked like [53] . Nevertheless, hominoid synapomorphies in the hand [26] , elbow [29] , ankle [27] , face [54] , dentition [1] and ontogenetic timing [55] of Proconsul provide solid support for the phylogenetic interpretation used here. Likewise, the intriguing differences in postcranial anatomy between Proconsul and Morotopithecus provide important evidence of variation in the Early Miocene, but do not necessarily imply that only one of these is a hominoid. Uncertainty surrounding the phylogenetic position of Proconsul notwithstanding, this genus remains a touchstone for understanding catarrhine and hominoid evolution based on the unprecedented number and quality of remains attributed to it. Regardless of whether the Proconsul lineage originated before or subsequent to the cercopithecoid-hominoid split, its morphology, adaptations and ecology provide information about an important stage in catarrhine evolution relevant to the origin of the Hominoidea [2] . The phylogenetic position of Dendropithecus is less contentious, although its precise relationships to other basal catarrhines are far from resolved. Dendropithecus is known from a number of cranial and postcranial remains, the latter due to the discovery in 1950 of four partial skeletons at the R3 site [23] . Initially, this primate was thought to represent a primitive ancestor of gibbons and siamangs [56] , but subsequent analyses demonstrated that it has a more conservative anatomy, similar in its locomotor repertoire to modern platyrrhines [2] . Today, most researchers place Dendropithecus outside of the crown catarrhines [1] , [2] , [57] , [58] , [59] , [60] , [61] , [62] , [63] , [64] , [65] , [66] , [67] . How to cite this article: Michel, L.A. et al. Remnants of an ancient forest provide ecological context for Early Miocene fossil apes. Nat. Commun. 5:3236 doi: 10.1038/ncomms4236 (2014).